A bio-inspired swellable microneedle adhesive for mechanical interlocking with tissue Achieving significant adhesion to soft tissues while minimizing tissue damage poses a considerable clinical challenge. Chemical-based adhesives require tissue-specific reactive chemistry, typically inducing a significant inflammatory response. Staples are fraught with limitations including high-localized tissue stress and increased risk of infection, and nerve and blood vessel damage. Here inspired by the endoparasite Pomphorhynchus laevis , which swells its proboscis to attach to its host’s intestinal wall, we have developed a biphasic microneedle array that mechanically interlocks with tissue through swellable microneedle tips, achieving ~3.5-fold increase in adhesion strength compared with staples in skin graft fixation, and removal force of ~4.5 N cm −2 from intestinal mucosal tissue. Comprising a poly(styrene)- block -poly(acrylic acid) swellable tip and non-swellable polystyrene core, conical microneedles penetrate tissue with minimal insertion force and depth, yet high adhesion strength in their swollen state. Uniquely, this design provides universal soft tissue adhesion with minimal damage, less traumatic removal, reduced risk of infection and delivery of bioactive therapeutics. Achieving significant levels of adhesion to soft tissues presents considerable challenges, especially when tissues are wet [1] , [2] . Chemical adhesives, such as cyanoacrylate, adhere strongly to tissues by a reactive exothermic covalent crosslinking reaction. However, these adhesives often cure too fast or too slowly and release toxic degradation products such as formaldehyde, leading to an intense inflammatory response [3] . While clinically utilized fibrin glue can effectively bond to wet tissue without a significant inflammatory response, it exhibits low strength of adhesion due to poor cohesive properties [4] , and can be challenging to apply as the polymerization time is difficult to control during placement. Alternatively, biocompatible hydrogel adhesives [5] , [6] that covalently bond to specific tissues can achieve a significant level of adhesion, yet their effectiveness depends on the presence of surface biomolecules with specific functional groups (e.g., NH 2 , SH or COOH). Therefore, the chemistry must be tailored for each tissue, and hydrogel adhesives do not adhere strongly to tissues such as skin. Also, it is critical to note that adhesives that rely on chemical bonding can easily be fouled in the presence of blood, thus compromising their efficacy in many surgical settings. For universal use, gold standard sutures and staples based on mechanical fixation are widely used [7] , [8] , [9] , however their placement can extend operating times as the tissue often must be manipulated before each pass of a suture needle. Sutures are difficult to place in small spaces (that is, during laparoscopic procedures) [10] , and do not work effectively for repair of many tissues including the dura mater [7] , urethral defects [8] and lung tissue [9] . While staples are typically quicker and easier to place than sutures, they can cause significant tissue damage, scarring, and excessive depth of tissue penetration can result in nerve and blood vessel damage [11] . Staples also pose a higher risk of developing a wound infection compared with sutures [12] . There are several unmet clinical needs for adhesives to affix connective tissues, including tendons and ligaments, to improve contact between tissues to reduce motion of tissue grafts, and to seal tissues for prevention of fluid (intestine) or air (lung) leaks. New adhesives are also needed to prevent formation of seromas following operations that create dead space between layers of tissue (for example, abdominoplasty), thus avoiding the need for drains that increase the risk of infection and potential necessity for reoperation [13] . A suitable platform approach to overcome the limitations of existing adhesives should ideally avoid the use of reactive chemistry, provide strong tissue adhesion in both normal and shear directions, be amenable to quick application, be simple to position over the target site, be removable (or degradable) with minimal tissue damage, provide adhesion to dynamic tissue surfaces while withstanding multiple extension/compression cycles, minimize the risk of infection and have the capacity to deliver therapeutics. Compared with glues, sutures and staples, tissue adhesive tapes have shown significant advantages including reduced procedure times, reduced scarring, ability to spread tissue forces over a larger surface area and enhanced tissue handling [14] , [15] , [16] . Additionally, adhesive tapes may be useful as an internal equivalent of a transdermal drug delivery patch to deliver drugs such as antibacterial, proregenerative or anti-inflammatory agents to target tissues. While barrier membranes and hernia meshes are routinely used clinically, these typically provide minimal adhesion, and often several sutures or tacks are used for fixation. Tape adhesives with hook-like protrusions have been developed, however their adhesion to tissue is fundamentally limited to surface entanglement without penetration of the tissue [17] . In seeking an optimal method of universal soft tissue adhesion with minimal tissue damage, we looked for inspiration from living organisms that have through the course of evolution adapted this function. Endoparasitic worms known as spiny-headed worms use a proboscis to penetrate through tissue. Species, such as Pomphorhynchus laevis, secure firm anchorage to the fish intestinal wall by expanding a bulb using retractor muscles at the base of the proboscis following penetration [18] . Using the adaptable morphology of the worm proboscis, we looked to create a structured biphasic microneedle (MN) with optimal characteristics for needle insertion and retention in tissue. Here we demonstrate a highly engineered MN with a shape change swellable tip that facilitates mechanical interlocking with tissue ( Fig. 1a ). This design minimizes the force needed for tissue penetration, as the smooth, cone-shaped needles can be inserted into tissue in a dry (stiff) state and do not include protruding barb features, associated with other proposed MN-based adhesive platforms [19] . Significant pull-out force can be achieved through the rapid increased cross-sectional area that occurs with swelling at the needle tips on contact with water (in tissue), leading to localized tissue deformation and subsequent interlocking. The bio-inspired MN adhesive showed high levels of adhesion with wet tissues, such as skin and intestine tissue, regardless of differences in surface texture. Additionally, strong fixation can be achieved in dynamic tissues during multiple cycles of movement and as increased pull-out forces are achieved via swelling within tissue, the soft MN tips (that is, reduced modulus) enable removal without significantly damaging the tissue. Furthermore, unlike stiff MNs that may break during removal from tissue, the modulus change due to swelling prevents breakage of the swollen MNs. 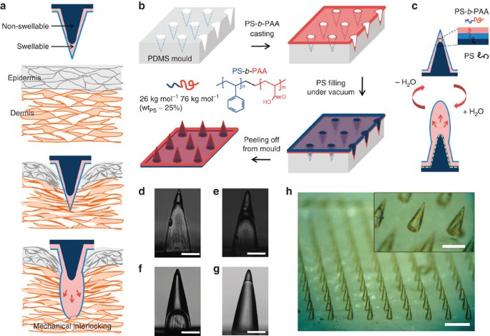Figure 1: Concept and fabrication of the bio-inspired microneedle (MN) adhesive. (a) Illustration showing mechanical interlocking of a water-responsive shape-changeable microneedle following penetration into a tissue. (b) Schematic showing the preparation of the double-layered MN array using a PDMS mould and showing the chemical structure of PS-b-PAA with PS weight fraction (wtPS) of 25% used for the swellable tip. (c) Cartoon showing the inner structure of double-layered MN and reversible water responsiveness. A thin hydrophobic film comprising the PS block covered the outer surface of the MN, likely due to the presence of the hydrophobic PDMS mould. During filling of the non-swellable PS core, PS chains likely entangle with the PS block at the interface (dashed line) between the swellable tip and PS core, providing interfacial adhesion to prevent delamination. (d–f) Side view images of hollow MN (without the PS core) with different PS-b-PAA filling fractions, including (d) 20%, (e) 40% and (f) 70% (height of PS-b-PAA layer compared with total MN height). These MNs were prepared by solvent-casting PS-b-PAA dissolved in DMF using different concentrations (d: 10 wt%,e: 18 wt% andf: 25 wt%). (g) Double-layered MN with a swellable tip (20% height fraction) following filling of the PS core. Scale bar, 200 μm. (h) Photograph of the double-layered MN array with density of 10 × 10 cm−2showing high-pattern fidelity. Scale bar, 1 mm. The PS-b-PAA tip is clearly distinguishable from the PS core as shown in the inset (Scale bar, 500 μm). Figure 1: Concept and fabrication of the bio-inspired microneedle (MN) adhesive. ( a ) Illustration showing mechanical interlocking of a water-responsive shape-changeable microneedle following penetration into a tissue. ( b ) Schematic showing the preparation of the double-layered MN array using a PDMS mould and showing the chemical structure of PS- b -PAA with PS weight fraction (wt PS ) of 25% used for the swellable tip. ( c ) Cartoon showing the inner structure of double-layered MN and reversible water responsiveness. A thin hydrophobic film comprising the PS block covered the outer surface of the MN, likely due to the presence of the hydrophobic PDMS mould. During filling of the non-swellable PS core, PS chains likely entangle with the PS block at the interface (dashed line) between the swellable tip and PS core, providing interfacial adhesion to prevent delamination. ( d – f ) Side view images of hollow MN (without the PS core) with different PS- b -PAA filling fractions, including ( d ) 20%, ( e ) 40% and ( f ) 70% (height of PS- b -PAA layer compared with total MN height). These MNs were prepared by solvent-casting PS- b -PAA dissolved in DMF using different concentrations ( d : 10 wt%, e : 18 wt% and f : 25 wt%). ( g ) Double-layered MN with a swellable tip (20% height fraction) following filling of the PS core. Scale bar, 200 μm. ( h ) Photograph of the double-layered MN array with density of 10 × 10 cm −2 showing high-pattern fidelity. Scale bar, 1 mm. The PS- b -PAA tip is clearly distinguishable from the PS core as shown in the inset (Scale bar, 500 μm). Full size image Bio-inspired MN array To create a stimulus responsive MN platform with low penetration force and strong adhesion, we pursued a double-layered MN design with selective localization of swellable material in the tip region. Following preferential distal swelling, each MN had both soft (outer) and stiff (inner) regions. In addition to having a MN platform comprising both swellable and non-swellable components, we sought to control the mechanical and water permeation properties of the swellable material, while promoting significant interaction between the soft outer layer and the stiff inner layer to prevent delamination. For this purpose, we considered an amphiphilic block copolymer (BCP) design that exhibits selective responsiveness to stimuli such as the presence of aqueous or organic solvents [20] , [21] . We envisioned that dual hydrophilic–hydrophobic properties of the outer layer would enable rapid absorption of water and promote intimate interaction with the non-swellable inner hydrophobic region. Block copolymers contain two or more chemically different polymers connected by covalent bonds that offer a means of combining the desirable characteristics of different polymers into a hybrid material [22] . The mechanical properties and swellability of the outer region of the MNs can be controlled by manipulating the overall average molecular weight of the polymer and the weight fraction of each block [20] , [23] . In this study, we chose a polystyrene- block -poly(acrylic acid) (PS- b -PAA) block copolymer as the swellable material and PS homopolymer as a non-swellable material. PAA is a well-known super-absorbent polymer used in several biomaterials-based strategies and in consumer products such as diapers that possesses COOH groups that quickly become ionized in the presence of water. In contrast, PS exhibits mechanical strength and structural integrity without swelling. As predicted, high volume expansion occurred when PAA was the major block component (over 70% in weight fraction). The mechanical robustness of the block copolymer could be strengthened by increasing the weight fraction of the PS block ( Supplementary Fig. S1 ). Interestingly, the stiffness of the block copolymer in its swollen state, with PS of ~25% weight fraction, approximates that of skin or intestine tissue ( Supplementary Fig. S1 ), which reduces the risk of underlying tissue damage without significantly compromising the interlocking mechanism. To permit rapid water penetration into the PS- b -PAA layer when the PS block preferentially assembles at the air-copolymer surface, we selected a PS block with a relatively low-molecular weight (<100,000 g mol −1 ) that minimizes interfacial surface area coverage due to short polymer chains. To achieve this, PS- b -PAA was prepared from the hydrolysis of polystyrene- block -poly( tert -butyl acrylate) (PS- b -P t BA) with number-average-molecular weights ( M n ) of 26,000 g mol −1 for PS and 128,000 g mol −1 for P t BA. Complete conversion of P t BA to PAA was confirmed by nuclear magnetic resonance (NMR) ( Supplementary Fig. S2 ). For functional testing in tissue, we selected swellable tips fabricated with PS- b -PAA with M n of 26,000 g mol −1 and 76,000 g mol −1 for PS and PAA, respectively, and a PS weight fraction of ~25%. As shown in Fig. 1a , b a double-layered MN array having water-swellable tips was fabricated by solvent-casting a PS- b -PAA solution in N, N- Dimethylformamide (DMF) on a PDMS (polydimethylsiloxane) mould with a 10 × 10 array of conical cavities within a 1 cm 2 area. Drying of the solvent prompted the formation of a thick film at the tip region of the conical cavity via capillary forces and a thin film on the remainder of the mould. To form the MN inner core and backing layer of the film, the PS homopolymer was melted on top of the continuous PS- b -PAA layer at 180 °C under vacuum. After cooling to room temperature, the double-layered conical MN array was carefully peeled from the PDMS mould. Macroscopically, the double-layered BCP MN exhibits a ‘needle-in-needle’ structure consisting of swellable outer PS- b -PAA layer and supporting PS inner core ( Fig. 1c ). Microscopically, the PS- b -PAA layer self-assembles into multiple phases whose location and properties are dependent on the interaction with the mould and air surface. To examine the composition of the swellable polymer surface at the air and PS core interfaces, we performed X-ray photoelectron spectroscopy (XPS) on PS- b -PAA films that were casted onto PS and PDMS substrates ( Supplementary Fig. S3 ). Given that the theoretical C/O ratio for PAA is 1.5, the C/O ratio at the surface of the PS- b -PAA layer on PDMS (14.9) and PS (22.3) suggests that PS was the dominant interfacial block. Thus, we speculate that a loosely packed PS film with a thickness of ~10 nm forms at the surface of the PDMS mould (air interface following removal from the mould) and modulates the rate of diffusion, preventing a rapid modulus drop caused by immediate water absorption, which would result in insertion failure of the BCP MN array. Furthermore, during filling of inner core by melted PS, the PS block in the PS- b -PAA layer can entangle with a PS homopolymer core and the COOH groups in the PAA chains thermally crosslink via intermolecular anhydride formation [24] , [25] . By varying the concentration of the casting solution, the height of the PS- b -PAA layer was controlled to be either 20, 40 or 70% of BCP MN height ( Fig. 1d–f ). Importantly, the PS base material completely filled the inner cores showing good contact with the PS- b -PAA layer ( Fig. 1g ). Figure 1h shows macroscale images of a double-layered BCP MN array with high-pattern fidelity having a density of 10 × 10 cm −2 , and having a swellable tip height of 20%, a MN base diameter of 280 μm and a MN height of 700 μm. An overall needle height of 700 μm was selected to ensure that the needle tip swelling would occur beneath the surface of the tissue (for example, thickness of epidermis is less than 100 μm at typical needle insertion sites) [26] and to minimize the penetration depth. Reversible shape change of a water-responsive swellable MN To visualize the real-time shape change of swellable BCP MN, we monitored the swelling behaviour immediately following insertion into a transparent agarose hydrogel (see Supplementary Fig. S4 for experimental setup). Once BCP MNs were inserted into the hydrogel (tip height ~40% of total MN height), the volume of the PS- b -PAA tip layer rapidly increased and reached ~60% of the maximum swollen state within 1 min. Subsequently, swelling equilibrated to a maximum swollen state within 10 min ( Fig. 2a and Supplementary Movie 1 ). The kinetics of water absorption of micron-sized PS- b -PAA were much faster than those of bulk material with mm-scale thickness ( Supplementary Fig. S1 ), which was likely the result of the high surface area per volume ratio for the MN tips and short water diffusion length. At equilibrium, the volume of PS- b -PAA MN layer had expanded to ~9 times its initial volume ( Supplementary Fig. S5 ). Volume expansion of BCP MN by swelling predominantly occurred in the tip region and swollen BCP MN interlocked with the hydrogel. The interlocked BCP MN could be removed from agarose gel without breakage or delamination. The swollen tips immediately began to deswell following retrieval from the hydrogel substrate and fully recovered to their original conical structure within 15 min ( Supplementary Fig. S6 and Supplementary Movie 2 ). 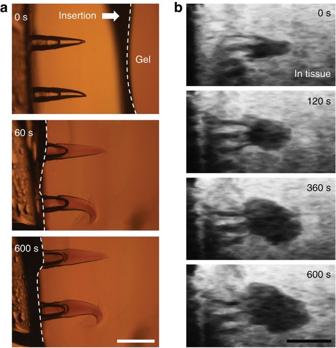Figure 2: Swelling of BCP MN following insertion into a hydrogel and muscle tissue. (a) Time-dependent swelling of the BCP MNs (40% swellable tip height fraction) following insertion into a 1.4 wt% agarose hydrogel (0, 60 and 600 s). (b) OFDI images showing swelling of the same BCP MNs following insertion into muscle tissue (0, 120, 360 and 600 s). Scale bar, 500 μm. Figure 2: Swelling of BCP MN following insertion into a hydrogel and muscle tissue. ( a ) Time-dependent swelling of the BCP MNs (40% swellable tip height fraction) following insertion into a 1.4 wt% agarose hydrogel (0, 60 and 600 s). ( b ) OFDI images showing swelling of the same BCP MNs following insertion into muscle tissue (0, 120, 360 and 600 s). Scale bar, 500 μm. Full size image When PS or PAA homopolymers were used as the MN tip material, they produced opposing results. The non-swellable PS MN was easily inserted into the hydrogel and freely removed without significant applied force, whereas the PAA MN did not penetrate the hydrogel because of low mechanical strength ( Supplementary Fig. S7 ). Although it is possible to make stiff PAA MN that can be inserted into hydrogel (or tissue) by crosslinking following harsh thermal treatment, pure PAA MN is also prone to delamination during removal of the MN due to poor interfacial adhesion with the backing layer. To verify the stimulus-responsive mechanical interlocking of the BCP MN in animal tissue, we utilized optical frequency domain imaging (OFDI) that is capable of providing non-invasive cross-sectional views of internal tissue structures to a depth of 1–2 mm with high resolution [27] . While the BCP MN inserted into muscle tissue showed less initial volume expansion rate compared with the agarose hydrogel, it reached the same final swollen state within 10 min ( Fig. 2b and Supplementary Movie 3 ). Interestingly, insertion into muscle tissue induced radial expansion of the BCP MN compared with axial swelling within the homogeneous agarose hydrogel. As observed within muscle tissue via OFDI, the swollen BCP MN formed a mushroom-shaped structure that provides a more favourable geometry to support mechanical interlocking with tissue. Firm adhesion of the swellable MN adhesive The adhesive properties of the BCP MN were evaluated by testing the normal adhesion strength of a 10 × 10 MN array (1 cm 2 cross-sectional area) on fresh cadaveric porcine skin. We investigated the effect of swelling-induced MN shape change on adhesion, compared with the adhesion of non-swellable PS MN ( Fig. 3a ). Adhesion of flat PS- b -PAA (BCP) and PS films were also measured. Both flat-surfaced BCP and PS films showed low adhesion strength to skin (<0.1 N cm −2 ). While, BCP MN and PS MN showed similar force versus displacement profiles during skin insertion ( Supplementary Fig. S8 ) and exhibited similar adhesion strength to skin immediately after insertion, after 10 min the maximum swollen state for BCP MN was achieved and the adhesive strength of the BCP MN dramatically increased. BCP MN with a swellable tip height of 20% (BCP MN (20%)) showed ~7 times higher adhesion strength (0.69±0.17 N cm −2 ) than PS MN adhesive (0.098±0.015 N cm −2 ). Furthermore, for BCP MN with a swellable tip height of 40% (BCP MN (40%)), the adhesive strength increased ~12-fold (1.23±0.26 N cm −2 ). However, MN with a swellable tip height of 70% (BCP MN (70%)) exhibited reduced adhesive performance ( Supplementary Fig. S9 ), likely due to a less favourable configuration for interlocking with tissue. No significant increase in adhesive strength was observed for the BCP MN for longer than 30 min swelling ( Fig. 3b ). For most intended uses, a short application time is desirable; therefore, the swelling time was standardized at 10 min for all additional experiments. 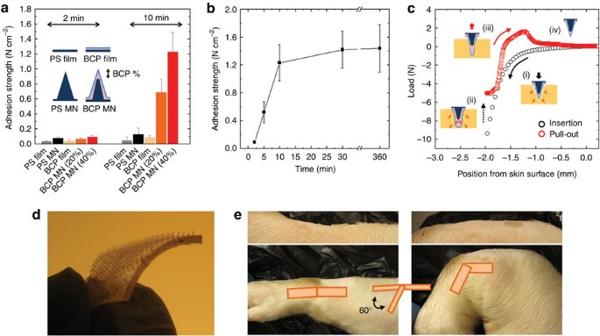Figure 3: MN adhesive firmly adheres to skin. (a) Normal adhesion strength for PS MN and BCP MN adhesives with 20 and 40% swellable tip height fractions following insertion into skin (2 and 10 min). Flat PS and PS-b-PAA films were used as controls. (b) Effect of swelling time within skin on adhesion for a BCP MN adhesive with a swellable tip height fraction of 40%. (c) Representative force-displacement curve during BCP MN insertion into, and removal from pig skin. (d) Photograph of flexible BCP MN adhesive (2 × 2 cm) prepared by using a thermoplastic elastomer as the base material (in place of PS). (e) Adhesion on a dynamic surface. Flexible BCP MN adhesives applied to shaved skin on top of the pig wrist joint showed firm attachment during ~100 cycles of bending motion. All error bars represent standard deviation. Figure 3: MN adhesive firmly adheres to skin. ( a ) Normal adhesion strength for PS MN and BCP MN adhesives with 20 and 40% swellable tip height fractions following insertion into skin (2 and 10 min). Flat PS and PS- b -PAA films were used as controls. ( b ) Effect of swelling time within skin on adhesion for a BCP MN adhesive with a swellable tip height fraction of 40%. ( c ) Representative force-displacement curve during BCP MN insertion into, and removal from pig skin. ( d ) Photograph of flexible BCP MN adhesive (2 × 2 cm) prepared by using a thermoplastic elastomer as the base material (in place of PS). ( e ) Adhesion on a dynamic surface. Flexible BCP MN adhesives applied to shaved skin on top of the pig wrist joint showed firm attachment during ~100 cycles of bending motion. All error bars represent standard deviation. Full size image The shape change adhesive mechanism of the BCP MN within porcine skin is shown in Fig. 3c . Following insertion into skin ( Fig. 3c(i) ), the tissue recoils and applies a mechanically compressive force against the BCP MN shaft. The position of the BCP MN is held fixed as the inserted BCP MN immediately swells in the presence of interstitial fluid and rapid volume expansion nears completion within 10 min, where the shape of the swollen tip stabilizes. The concentrated volume expansion at the tip of the BCP MN ( Fig. 3c(ii) ) leads to an arrow-head-like structure facilitating mechanical interlocking with the tissue. Removal of the BCP MN from the skin can be safely performed without fracture or delamination due to the deformability of the swollen tip and strong interfacial interaction between the swollen layer and base material ( Fig. 3c(iii) ). Significant adhesive strength was maintained even at high levels of strain between BCP MNs and skin until BCP MNs are fully removed from the skin, indicating that the BCP MN exhibits high adhesion energy. Owing to the reversible responsiveness in water ( Fig. 3c(iv) ), the swollen BCP MNs quickly return to their original conical structure after removal. Following recovery of shape and stiffness ( Supplementary Fig. S10 ), the BCP MN exhibited reversible adhesive properties during multiple swelling/deswelling cycles; therefore it is possible that the BCP MN could be reused following sterilization by ethanol or autoclave treatment. We compared the adhesive strength of the BCP MN with currently used commercial pressure-sensitive adhesive bandages on semi-dry and wet porcine skin surfaces ( Supplementary Fig. S11 ). While commercial bandages show higher adhesive strength on dry skin surfaces compared with the BCP MN adhesive, the adhesive strength of commercial bandages on wet skin decreased by more than 50%. However, BCP MNs showed similar adhesive strength regardless of the presence of water on the tissue surface. To demonstrate the versatility of the BCP MN adhesive, the stiff PS base material was substituted for a flexible thermoplastic PS-based elastomer ( Fig. 3d ). The flexible BCP MN adhesive (Flex BCP MN) with 10 × 10 array in a 1 cm 2 was applied to a wet skin surface on top of a pig wrist joint that was cycled through an angle of ~60° to stretch and compress the tissue. Flex BCP MNs maintained strong attachment without migration during 100 cycles of bending motion ( Fig. 3e and Supplementary Movie 4 ). MN adhesive for use in skin graft fixation With regard to potential immediate applications of BCP MN adhesives, we envision fixation of skin grafts as a strong candidate. Skin grafts are often employed for closure of open wounds as a result of burns, trauma or surgical resections [28] , [29] . For successful engraftment, continuous contact between the skin graft and underlying tissue is essential to assure graft survival by directed diffusion of wound bed nutrients as well as to prevent haematoma or seroma formation [30] . Sutures or staples applied to the perimeter of the skin graft represent the current standard of care, and frequently this results in separation between the tissue layers, as direct fixation only occurs along the periphery of the wound. Furthermore, fixation by staples is not rigid enough to avoid motion and shear resulting frequently in partial or complete loss of the graft. The likelihood of failure is diminished by secondary dressings, and grafted body part immobilization. From dye diffusion tests, we found that staples provided a surface contact area of ~50% between the skin graft and underlying hydrogel, and that the staples produced significant damage to the hydrogel during insertion and removal ( Fig. 4a ). In contrast, the BCP MN adhesive showed continuous contact of ~100% with minimal damage to the hydrogel ( Fig. 4b ). As marked by an arrow in Fig. 4a , the depth of penetration (~3 mm) of staples causes significant tissue damage and results in a higher risk of bacterial infiltration. In adhesion testing, although stapled skin grafts did not fully detach from underlying tissue during pull-off, central regions of the skin grafts were separated due to low adhesion strength ( Fig. 4c ). Skin grafts fixed using the BCP MN adhesive on muscle tissue showed significantly higher adhesive strength (0.93±0.23 N cm −2 ) than stapled skin grafts (0.28±0.11 N cm −2 ) and non-fixed skin grafts (0.22±0.09 N cm −2 ) ( Table 1 ). The attachment was maintained following an elongation of ~4 mm, which is more than five times the height of the BCP MN ( Fig. 4d ). To prevent the accumulation of fluid at the interface between BCP MN adhesive and skin graft, drainage holes can easily be placed within the backing material of the adhesive array ( Supplementary Fig. S12 ). An ideal tissue adhesive should also provide a biological barrier to reduce the risk of surgical site infection. In the case of staple fixation, stress concentrations localized around the staple legs can cause excessive tearing of a skin graft and produce a larger hole than a diameter of the staple ( Fig. 4e ). Staple holes serve as a pathway for bacterial infiltration [12] and as expected, Escherichia coli ( E. coli ) transformed to express the green fluorescent protein (GFP), infiltrated through the staple holes and formed colonies ( Fig. 4f ). For the BCP MN adhesive, the interlocked and swollen MNs tightly seal the punctured holes, thus preventing the physical passage of microorganisms ( Fig. 4g ). The BCP MN adhesive was removed without a significant damage to the agar layer (left image in Fig. 4h ) and GFP signal was not detected in the agar plate placed beneath the incised skin grafts covered by the BCP MN (right image in Fig. 4h ). As a result of the non-permeable backing layer and tight sealing of the punctured holes by the swollen MNs, the BCP MN adhesive effectively prevents the infiltration of bacteria, which is a main cause of infection. 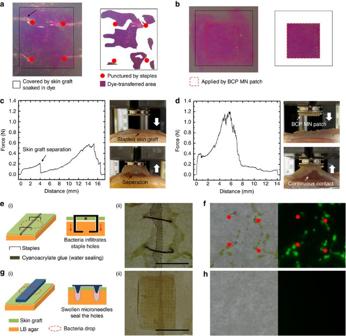Figure 4: MN adhesive achieves effective fixation of skin grafts and resists bacterial infiltration. (a,b) Comparison of the contact area between a skin graft and tissue-like hydrogel (4 wt% agarose gel) after (a) applying staples and (b) a BCP MN adhesive. Staples showed less contact area between the skin graft and underlying hydrogel and on removal induced significant damage to the underlying hydrogel (region marked by arrow inFig. 4a), while the BCP MN adhesive showed continuous contact ~100% with minimal damage to the hydrogel. (c,d) Force-displacement profiles and photographs acquired during pull-off tests of skin graft on muscle tissue fixed by (c) staples and (d) BCP MN adhesive. While the stapled skin graft was easily separated from the underlying muscle with a low pull-off strength, the BCP MN adhesive provided continuous contact between the skin graft and muscle tissue via mechanical interlocking with underlying muscle tissue. (e–h) Comparison of the bacterial barrier property of incised skin grafts following application of (e,f) staples and (g,h) a BCP MN adhesive. (e(i)) Cartoon illustrating the primary site of bacterial infiltration through the gaps between staple legs and skin grafts. (e(ii)) A photograph showing stapled skin grafts after bacteria infiltration; cyanoacrylate glue was used to tightly seal the incised region (dark area outlined by dotted black line). (f) GFP-expressingE. colicolonies formed near deep staple holes (marked by red dots) where skin grafts did not appose the underlying agar layer (left, bright field image). The infiltration ofE. colithrough the staple holes was confirmed by green fluorescence (right, fluorescent image). (g(i)) Cartoon showing bacterial barrier resistance of the BCP MN adhesive resulting from tight sealing of holes by swollen MNs. (g(ii)) Photograph of the BCP MN adhesive applied on the incised skin grafts. (h) BCP adhesive prevented bacterial infiltration (left, bright field image) with minimal damage and (right, fluorescent image) no green fluorescence was detected on the agar plate. Scale bar, 1 mm. Figure 4: MN adhesive achieves effective fixation of skin grafts and resists bacterial infiltration. ( a , b ) Comparison of the contact area between a skin graft and tissue-like hydrogel (4 wt% agarose gel) after ( a ) applying staples and ( b ) a BCP MN adhesive. Staples showed less contact area between the skin graft and underlying hydrogel and on removal induced significant damage to the underlying hydrogel (region marked by arrow in Fig. 4a ), while the BCP MN adhesive showed continuous contact ~100% with minimal damage to the hydrogel. ( c , d ) Force-displacement profiles and photographs acquired during pull-off tests of skin graft on muscle tissue fixed by ( c ) staples and ( d ) BCP MN adhesive. While the stapled skin graft was easily separated from the underlying muscle with a low pull-off strength, the BCP MN adhesive provided continuous contact between the skin graft and muscle tissue via mechanical interlocking with underlying muscle tissue. ( e – h ) Comparison of the bacterial barrier property of incised skin grafts following application of ( e , f ) staples and ( g , h ) a BCP MN adhesive. ( e (i)) Cartoon illustrating the primary site of bacterial infiltration through the gaps between staple legs and skin grafts. ( e (ii)) A photograph showing stapled skin grafts after bacteria infiltration; cyanoacrylate glue was used to tightly seal the incised region (dark area outlined by dotted black line). ( f ) GFP-expressing E. coli colonies formed near deep staple holes (marked by red dots) where skin grafts did not appose the underlying agar layer (left, bright field image). The infiltration of E. coli through the staple holes was confirmed by green fluorescence (right, fluorescent image). ( g (i)) Cartoon showing bacterial barrier resistance of the BCP MN adhesive resulting from tight sealing of holes by swollen MNs. ( g (ii)) Photograph of the BCP MN adhesive applied on the incised skin grafts. ( h ) BCP adhesive prevented bacterial infiltration (left, bright field image) with minimal damage and (right, fluorescent image) no green fluorescence was detected on the agar plate. Scale bar, 1 mm. Full size image Table 1 Tissue adhesion for skin grafts fixed by BCP MN adhesive and staples. Full size table While the micron-sized puncture marks created after removal of the MNs from the wound could serve as a source of infection, it has been reported that the skin recovers its barrier function within a few hours following MN removal [31] . The disappearance of puncture marks was confirmed within 1 h of removal of the swellable MN adhesive ( Supplementary Fig. S13 ). In addition, it has been reported that microbial penetration through the holes created by MNs is minimal [32] . Considering its rapid and long-term adhesion, this superior bacterial barrier provided by the BCP MN adhesive could reduce the risk of infection to open wounds including burn tissue. Firm adhesion of the MN adhesive to intestinal tissue To evaluate the capacity for BCP MN adhesives to be used to seal intestine tissue, which may be useful to prevent leaks following gut anastomosis procedures, we examined adhesion to the outer serosal surface ( Fig. 5a ) that is a relatively smooth surface (roughness of several micrometres) and inner wrinkled mucosal surface (roughness on the sub-mm scale) that is covered by a sticky mucin layer ( Fig. 5b ). The non-swellable PS MN adhesive applied to the outer surface of the intestine tissue ( Fig. 5c ) showed an adhesive strength of 0.48±0.18 N cm −2 , whereas a swellable MN adhesive with a PS base (BCP MN) showed an adhesive strength of 1.62±0.17 N cm −2 . Interestingly, the BCP MN adhesive exhibited an adhesive strength of 3.83±1.35 N cm −2 to the inner mucosal surface, possibly resulting from non-covalent interactions with mucin. Moreover, the Flex BCP MN showed further improvement in adhesive strength to the mucosal surface, up to 8 N cm −2 (mean value: 4.53 N cm −2 ). The enhanced adhesion of the Flex BCP MN on the mucosal surface may result from increased intimate contact during removal that may be facilitated by increased absorption of energy by the flexible backing material. The BCP MN adhesive appears to achieve adhesion to tissues that cannot be achieved effectively using conventional tape-based approaches [33] . As shown in Fig. 5d , inserted PS MNs into the outer surface of intestine tissue showed an average maximum torque of 0.85±0.28 Ncm during torsion tests, through a 60° angle of rotation. After removing PS MNs from the tissue, it was observed that ~30% MNs remained broken. When the PS MNs were exposed to 100° of rotation before removal from tissue, they showed a higher maximum torque (1.22±0.41 Ncm) and nearly all tips or whole bodies were broken ( Fig. 5e ). Comparatively, less than 5% of the BCP MN and none of the Flex BCP MN were broken following 60° of rotation, and less than 5% of Flex BCP MN were broken following 100° of rotation ( Fig. 5d ). Interestingly, puncture marks resulting from the BCP MN insertion into tissue disappeared within 2 h of removal ( Supplementary Fig. S14 ). 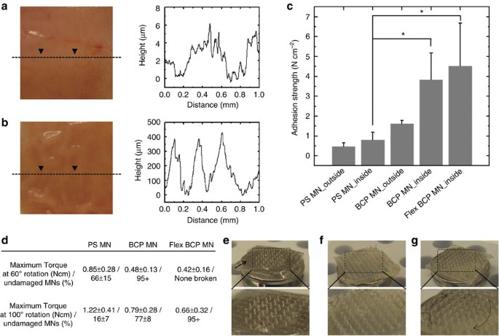Figure 5: MN adhesive firmly attaches to wet intestine tissue. (a,b) Photographs from (a) outer and (b) inner (mucosal) surfaces of pig intestine tissue and corresponding depth profile showing topographical roughness. (c) Adhesion strength for PS MN (non-swellable) and swellable BCP MN adhesives with a rigid and flexible base following insertion into mucosal and serosal intestine surfaces. The asterisk indicates statistical significance withP<0.05 (analysis of variance with post-hoc Tukey’s honestly significant difference test). Error bars represent standard deviation. (d) Following penetration into the outer surface of intestine tissue and application of 60° or 100° of rotation, significant damage to PS MN was observed (broken MN), while BCP MN and Flex BCP MN exhibited significantly reduced MN breakage. (e–g) Photographs for tilted view of MN arrays after torsion test of 100° rotation using (e) PS MN, (f) BCP MN and (g) Flex BCP MN adhesives. The tips or entire PS MNs were broken by torsional stress (especially at the edges of the patch marked by arrow (e)), yet BCP MN with rigid and flexible bases showed high resistance to torsional stress by bending in the direction of the shear force (marked by arrows in (g)). Figure 5: MN adhesive firmly attaches to wet intestine tissue. ( a , b ) Photographs from ( a ) outer and ( b ) inner (mucosal) surfaces of pig intestine tissue and corresponding depth profile showing topographical roughness. ( c ) Adhesion strength for PS MN (non-swellable) and swellable BCP MN adhesives with a rigid and flexible base following insertion into mucosal and serosal intestine surfaces. The asterisk indicates statistical significance with P <0.05 (analysis of variance with post-hoc Tukey’s honestly significant difference test). Error bars represent standard deviation. ( d ) Following penetration into the outer surface of intestine tissue and application of 60° or 100° of rotation, significant damage to PS MN was observed (broken MN), while BCP MN and Flex BCP MN exhibited significantly reduced MN breakage. ( e – g ) Photographs for tilted view of MN arrays after torsion test of 100° rotation using ( e ) PS MN, ( f ) BCP MN and ( g ) Flex BCP MN adhesives. The tips or entire PS MNs were broken by torsional stress (especially at the edges of the patch marked by arrow ( e )), yet BCP MN with rigid and flexible bases showed high resistance to torsional stress by bending in the direction of the shear force (marked by arrows in ( g )). Full size image The swellable MN adhesive presented here provides a new platform for adhesion based on mechanical interlocking. It harnesses a water based swelling mechanism that responds quickly and is reversible. While we chose PS and PAA as our materials in this proof-of-concept study, the strategy described herein could be applied using many other polymers. Conventional polymer-based MN systems are composed of relatively stiff materials so that they can penetrate tissue without deformation. However, this can often lead to brittle fracture of MNs when they are subjected to dynamic tissues. As our MN system is biphasic and becomes more ductile during the swelling process, we hypothesized that our system has a distinct advantage compared with other systems in this regard. As presented here, 100% of MNs remained intact regardless of the tissue type when swollen MNs with stiff or flexible cores were removed from the inserted tissues in the normal direction. In addition, the resistance of MNs to torsion-induced shear stress is compelling. Although it is difficult to quantify the exact levels of shear stress generated in this approach due to the complex interfacial geometry, at significant levels of shear strain (induced by 60° of rotation) 100% of Flex BCP MNs remain intact, while ~1/3 of PS MNs fracture. Considering previous achievements with MN-based drug delivery, it is expected that the MN adhesive could provide a dual function enabling a firm attachment and efficient drug permeation. This strategy would be especially useful for skin graft fixation, which requires intimate contact between the skin graft and the underlying wound bed over the entire surface area of the wound during movement, and a necessity to deliver medications such as anti-inflammatory/anti-scarring agents, antibiotics and bioactive peptides directly to the wound bed. As drugs can easily be loaded into the swellable tips during swelling, within an agent-doped solution (followed by deswelling to return to a stiff state), BCP MN adhesive can administer multiple types of agents directly into the wound microenvironment in a minimally invasive manner. To verify the potential use of the swellable MN for delivery of drugs, we loaded BCP MN with triamcinolone acetonide (TACA), a steroid with anti-scarring and anti-inflammatory properties, by allowing them to swell in a TACA solution. The BCP MN adhesive (100 MNs in 1 cm 2 ) showed ~70% release of TACA over the course of 1 day in deionized (DI) water, with the remaining TACA released over several days. Additionally, towards potential delivery of biologics, we showed that the BCP MN swellable tips could encapsulate fluorescein isothiocyanate-labelled dextran ( M w : 2,000,000 Daltons) with a hydrodynamic diameter of ~100 nm during the swelling process ( Supplementary Fig. S15 ). PS and PAA were chosen as components of our swellable MN system given their established potential to exhibit only a minimal inflammatory response on implantation [34] , [35] . While we envision the approach could be employed with biodegradable materials, diffusion-based drug delivery through the swollen non-degradable MN is controllable and likely useful for short-term applications. While a change in the local acidic environment during the swelling process of PS- b -PAA could stimulate an inflammatory reaction, a relatively minor change in pH (7.3–6.8) of PS- b -PAA is observed compared with the PAA homopolymer (7.3–3.4) ( Supplementary Fig. S16 ). As highlighted by Banga et al . [36] , MN-based systems for drug delivery are largely analogous to the use of hypodermic syringes, with specific advantages associated with minimal user training and lower or no risk of injury to the user and patient. While there are regulatory issues associated with medication linked to the delivery material, in our MN system the only material that remains in the tissue on removal of the MN is the loaded drug; thus reducing the potential for a chronic foreign body response. In conclusion, we have demonstrated a new bio-inspired tissue adhesive platform governed by shape change-mediated mechanically interlocking MNs. This MN exhibits universal adhesion to soft tissues regardless of surface chemistry and it mechanically interlocks with tissues without significant damage while providing an effective barrier to bacteria. As the BCP MN can easily encapsulate model drugs, the MN adhesive may serve as an effective drug delivery vehicle to enhance the penetration of drugs into tissue. Owing to its capacity to conform to tissues with a broad range of surface textures, the BCP MN system has the potential for use in a wider range of medical applications than current tape-based adhesives. Fabrication of the MN array patch PS- b -PAA was prepared by hydrolysis of PS- b -P t BA (0.5 g, M n : 26–128 k, Polymer Source) in dry dichloromethane (20 ml) with trifluoroacetic acid (1.2 molar equivalent compared with tert -butyl ester groups) as a catalyst for 48 h. Then, PS- b -PAA was precipitated into hexane, filtered, and washed several times to remove any trace of the catalyst. Hydrolysis was confirmed by NMR ( Supplementary Fig. S2 ). The number-average-molecular weight ( M n ) of PS- b -PAA used for the swellable polymer was 26 kg mol −1 for PS and 76 kg mol −1 for PAA blocks. PS- b -PAAs with different compositions were also prepared by hydrolysis of PS- b -P t BAs ( M n : 19–729 k (PDI:1.23) and 24–36 k (PDI:1.09), Polymer Source) as described above. A female PDMS mould for the MN array (10 × 10) of 1 cm 2 was prepared using photolithography and moulding techniques as previously reported [37] . Briefly, to fabricate a female master mould, 1-mm-thick SU 8 film was spin-coated onto a Si wafer and exposed to ultraviolet light (365 nm, 10 W cm −2 ) through a chrome mask patterned with 300 μm diameter dots. The ultraviolet exposure was performed at an angle of 20° on a rotating stage at 10 r.p.m. for 450 s. After developing, each conical cavity was 700 μm deep with a base diameter of 280 μm and tip radius of 10 μm. Tip-to-tip spacing between cavities was 950 μm. Female PDMS (Sylgard 184, Dow corning) moulds were obtained from male PDMS moulds cast from the female master mould. The first layer of the MN patch was prepared by solvent casting the PS- b -PAA dissolved in DMF for 48 h followed by degassing, and the mass of material in the MN tips was controlled by altering the concentration of casting solution. To fabricate double-layered MN, PS pellets ( M w : 100 k, PDI: 1.06, Polysciences) were melted on solvent-casted PS- b -PAA at 180 °C and then stored under vacuum for 4 h. After cooling to room temperature, double-layered MN arrays (BCP MN) were gently peeled from the mould. Single PS MN arrays were prepared by melting PS pellets in moulds at 180 °C under vacuum for 4 h. To fabricate a flexible MN patch (Flex BCP MN), styrene-isoprene-styrene copolymer (weight fraction of PS: 22%, Aldrich) was used in place of the PS second layer via melt casting on the underlying PS- b -PAA layer. To fabricate flat PS- b -PAA substrates for adhesion testing, PS- b -PAA was solvent casted on PDMS flat substrates (1 × 1 × 0.5 cm 2 well) for 48 h and then PS was filled by melt casting at 180 °C for 4 h. Flat PS samples were prepared by melt casting flat PDMS moulds with PS. The morphology of MN was examined with optical microscopy (E100, Nikon). Swelling and mechanical properties of PAA homopolymer and PS- b -PAAs PAA homopolymer (Mv: 450,000, Aldrich) and PS- b -PAAs were dissolved in DMF and cast in PDMS wells followed by drying for 7 days at room temperature in a fume hood. Casted films with a thickness of ~1 mm were cut using a 4-mm diameter biopsy punch and the punctured discs were subsequently dried at 180 °C for 4 h. After cooling at room temperature, discs were immersed in phosphate-buffered saline (PBS) buffer (pH 7.4) at room temperature. The mass of each sample was measured after removal of surface water at each time point. The compressive modulus of polymer samples was characterized after they reached their maximum swollen state. The samples placed in a water bath were subjected to a compressive axial load at a strain rate of 0.5 mm min −1 using an eXpert 760 mechanical tester (ADMET) at room temperature. The load-displacement data were transformed to stress-strain plots. The slope of a linear fit for 5% strain was used as a measure of the compressive modulus. The mean compressive modulus was measured from n =5 different samples. XPS measurement to examine the surface composition of PS- b -PAA films To examine the surface composition of the swellable BCP MN at the PDMS (air interface following removal from the mould) and PS core interfaces, we prepared PDMS and PS substrates. For the PS-grafted surface, a hydroxyl-terminated polystyrene (PS-OH, M n =10,000 g mol −1 , PDI=1.08, Polymer Source) solution in toluene was spin-coated onto Si wafer, cleaned by immersion for 20 min at 85 °C in a piranha solution (1:4 mixture of 30% H 2 O 2 and concentrated sulphuric acid). The grafting of PS on the Si substrate was completed by annealing the samples at 170 °C under vacuum for 1 day. Unbound PS-OHs were removed by sonication in toluene before use. The thickness of the PS brush was measured to be 7–8 nm by using an ellipsometer (JA Woollam company, Model WVASE32). A PS- b -PAA (26 k–76 k) solution in DMF was cast on the PDMS and the PS-grafted Si wafer for 2 days and then dried at 180 °C for 4 h. After cooling in air to room temperature, the prepared films were peeled from the substrates using double-sided tape. Elemental analysis of the bottom surface of the PS- b -PAA film that contacted the PDMS or PS brush was examined by XPS (Surface Science, model SSX-100) with a monochromatic Al Kα X-ray source. Visualization of BCP MN shape change by swelling To observe the swelling behaviour of the MN, one row of MNs was cut from an array attached to a metal specimen, and swelling of the MN was recorded using inverted microscope after insertion into a 1.4 wt% agarose hydrogel ( Supplementary Fig. S4 ). Shape change of BCP MNs by swelling in animal tissue was assessed using OFDI [27] , a second-generation optical coherence tomography technology. In short, light from a wavelength-swept laser source (1,220–1,360 nm) was split into reference and sample arm by means of a fibreized interferometer. The sample light was focused into a spot with 30 μm waist radius and scanned over the tissue. The reflected light was recombined with the reference signal before detection, digitized, and reconstructed to yield the depth resolved scattering profile at each scanning position. BCP MNs were inserted frontally into a cube of chicken muscle, close to the top tissue surface to enable imaging with OFDI. An area of 5 × 3 mm, consisting of 1,024 × 512 depth profiles, was scanned at a 2-min interval. The reconstructed cross-sectional images showed signal void regions in the area of the BCP MNs, contrasted by a high scattering signal from the surrounding tissue. Minimum intensity projections along the lateral direction of MNs were taken after smoothing the tomograms to reduce speckle and provided a clear view of the shape profile of MNs. Measurement of adhesion force with porcine skin Full-thickness porcine cadaver skin was stored frozen and cut into ~2 × 2 cm patches followed by immersion in PBS for 1 h. For semi-dry adhesion tests, water was removed from the surface of porcine skin with blotting paper and the skin was dried on blotting paper for several minutes until 10–20% of the absorbed water was removed. For wet adhesion testing, 200 μl of PBS buffer was spread across the surface of porcine skin before adhesion tests. Normal adhesion tests for samples with an area of 1 cm 2 were performed using an eXpert 760 mechanical tester (ADMET) with custom-fabricated stainless steel tissue grips and a 50 N load cell. This methodology was selected to enable comparison with the adhesive performance of staples. A flat section of skin tissue was affixed using cyanoacrylate glue to a test fixture (that is, pin mount stub with diameter of 25.4 mm) and mounted within the lower grips at the base of the mechanical tester. The MN (10 × 10 MNs array in 1 cm 2 ) or flat patch were glued onto the opposing test fixture and fixed between the upper grips of mechanical tester. Test samples were applied to tissues with 10 N of preload at 100 mm min −1 , and held in position for 2, 5, 10, 30 min or 6 h. Samples were displaced at a rate of 1 mm min −1 and the force was recorded. Dynamic adhesion testing was conducted on the shaved wrist of a pig following euthanasia. To ensure the surface was wet before testing, 1 ml of PBS buffer was spread over the skin before applying a MN patch. The degree of local skin elongation while moving the wrist from extension to maximum flexion was determined. A Flex BCP MN array with 10 × 10 MN in 1 cm 2 was adhered by applying manual compression for 10 min. The pig wrist was then subjected to dynamic testing (extension to maximum flexion, back to extension) through 100 cycles to determine its fixation ( Supplementary Movie 4 ). Measurement of contact area and adhesion force Unmeshed porcine skin grafts with a thickness of 200 μm were obtained from the back of postmortem pigs using a dermatome immediately after euthanasia, in accordance with animal health and welfare policies. They were kept in Dulbecco’s modified Eagle medium (DMEM) at 4°C and used within 2 weeks of harvest. To examine the contact area between the adhesive patch and underlying tissue, dye diffusion tests were performed. After application of the MN patch or staples, the skin graft (1.5 × 1.5 cm) was presoaked in 0.1 wt% solution of Rhodamine dye for 10 min and transferred onto a 4 wt% agarose hydrogel after removal of the excess dye solution. Staples or a BCP MN adhesive were applied to fix the skin graft onto the hydrogel for 2 min. The contact area was determined by the dye-transferred region via image analysis software. For adhesion tests, skin grafts were cut into 1.5 × 1.5 cm patches and placed on a flat section of muscle tissue (2.5 × 2.5 cm) that had been affixed using cyanoacrylate glue to the bottom test fixture. The MN patches (10 × 10 MNs array in 1 cm 2 ) were glued to the top fixture of the mechanical tester and applied to the underlying tissues with 20 N of preload at 150 mm min −1 and held in position for 10 min. Samples were then displaced at a rate of 1 mm min −1 and the force was recorded. To compare adhesion force between the stapled skin graft and underlying muscle tissues, staples were applied to the perimeter of the skin graft with spacing of 1.3–1.5 cm using a skin stapler (Reflex One, CONMED). For experiments with the MN patch, the same preload (20 N) was used and a pin mount stub with a diameter of 12 mm was applied to the stapled skin graft. For the duration of all experiments, the tissue was kept moist with PBS. In vitro assessment of bacterial infiltration BL21(DE3) competent E. coli (New England Biolabs) was transformed with pFluoroGreen (EDVO-Kit 223, EDVOTEK) and cultured on ampicillin and isopropyl-β- D -thiogalactoside (IPTG) supplemented LB agar plates. A GFP-positive colony was picked to inoculate a 10 ml standard LB broth supplemented with ampicillin and IPTG. The GFP-expressing E. coli was cultured overnight at 37 °C and was diluted by 10 3 -fold into PBS buffer. This dilution yielded an inoculum of ~2 × 10 4 c.f.u. ml −1 . To prepare LB agar plates, LB agar medium powder (MP Biomedicals, LLC) was added to DI water and autoclaved at 121 °C for 15 min. After cooling to 50 °C, 15 ml of molten agar was supplemented with ampicillin and IPTG, poured into sterile Petri dishes (100 × 15 mm) and allowed to solidify. A 50 μl solution of bacteria (~1,000 cells) was pipetted onto the centre of the incised skin grafts (250 μm thick) placed on LB agar plate after applying staples or the BCP MN adhesive. To investigate the effect of staple holes on bacteria infiltration, the interface of two incised skin grafts was tightly sealed using cyanoacrylate glue before stapling. Testing plates were incubated at 37 °C for 24 h and were observed for the growth of GFP-expressing E. coli to examine the bacterial barrier resistance of the incised skin grafts closed by a BCP MN adhesive or staples ( n =3). Measurement of adhesion and torsional force with porcine small intestine Fresh intestine tissue was rinsed with PBS buffer several times and then cut into~2 × 2 cm patches. Surface water was removed with blotting paper while mucin remained on the inner surface of the intestine. Topography for the inner and outer surface of intestine tissue was measured by using a depth profiler (Sloan Dektak II) after freezing the tissue at −20 °C. Normal adhesion tests were conducted using the same experimental setup for porcine skin. For the duration of all experiments, the tissue was kept moist with PBS. The mean adhesion force was measured from n =5 different samples. Torsion tests were conducted using a biaxial transducer followed by the same experimental procedures used for the normal adhesion test. Samples inserted into tissue were rotated at a rate of 0.5 degree s −1 by 60 or 100 degree, and the force was recorded. Following the torsion test, breakage of MN was examined via macroscopic images. Controlled release of drugs from swellable tips of BCP MN adhesive Triamcinolone acetonide (TACA, Fluka) was loaded in the tips of BCP MN patch (100 MNs in 1 cm 2 ) via swelling in a TACA solution (4 ml) of 1 mg ml −1 dissolved in methanol. Following 30 min incubation, the BCP MN patch was washed by dipping in DI water, excess water on the surface of the needles was removed, and then the patches were dried at room temperature for 1 h. Drug-loaded BCP MN patches were placed into 6 ml of fresh DI water to examine the release of encapsulated TACA. A quantity of 0.6 ml of the solution was sampled at each time point, and 0.6 ml of the fresh DI water was replaced. The amount of released TACA was determined by HPLC system (Agilent 1100 series) with C18 column (5 μm) (250 × 4.6 mm ID, Agilent Eclipse XDB-C18) at 240 nm with an Agilent G1314A detector. Peak identification was achieved based on the comparison of retention times of compounds within standard solutions using ChemStation software (Agilent Technologies). Statistics Unless otherwise stated, all experiments were performed using at least five samples per group and the data presented are representative of five independent experiments. For multiple comparisons, analysis of variance was performed with the Tukey’s honestly significant difference test at significance levels of 95%. Error bars in bar graphs represent the standard deviation. How to cite this article: Yang, S.Y. et al . A bio-inspired swellable microneedle adhesive for mechanical interlocking with tissue. Nat. Commun. 4:1702 doi: 10.1038/ncomms2715 (2013).